Efficient selective and atom economic catalytic conversion of glycerol to lactic acid The availability of glycerol is rapidly increasing due to the expanding biodiesel industry, which produces this polyol as the main waste material. Several value-added chemicals have been synthesized using glycerol as a feedstock; however, the conversion of glycerol to lactic acid has been investigated to a lesser extent despite the numerous and novel uses of lactic acid. We report a family of iridium complexes as the first homogeneous catalysts for the conversion of glycerol to lactic acid. These have higher activity and selectivity than the previously reported heterogeneous systems. In addition, hydrogen gas is generated as a useful byproduct. Unlike prior systems, the reactions can be performed in air, under mild conditions and without solvent. Our method has even been applied to samples of crude glycerol waste derived from the biodiesel industry without prior purification, albeit with somewhat lower activity while maintaining the same high selectivity. The sustainable and environmentally sound use of natural resources is currently a major challenge in chemistry. In this context, biodiesel has emerged as an attractive fuel due to its environmental benefits, its capacity to overcome the dependence on foreign petroleum and the fact that it is manufactured from renewable resources [1] . Biodiesel is a rising alternative to fossil fuels, but its production will entail an increase in the production of glycerol as the main byproduct (~10 wt%). This offers promising opportunities for upgrading this waste material [2] , [3] . A number of catalysts, some homogeneous but mostly heterogeneous, have been employed to convert glycerol to several value-added products [4] , [5] , [6] such as propanediols [7] , [8] , acrolein [9] , [10] , dihydroxyacetone (DHA) [11] , [12] , [13] , glyceric acid [14] , [15] , cyclic acetals [16] or epichlorohydrin [17] , [18] , [19] . However, the conversion of glycerol to lactic acid (LA) has been less thoroughly explored despite its numerous applications [20] . LA is a platform chemical for the production of the biodegradable polyester, poly(lactic acid) (PLA), as well as a feedstock for the synthesis of green solvents and a broad variety of valuable commodity chemicals. LA is also directly employed in the pharmaceutical, food and detergent industries. Sugar fermentation accounts for over 90% of the current LA production; however, this method has several important drawbacks, such as limited space–time yield, poor productivities (grams of LA per liter of reaction mixture per hour) due to the need for dilute glycerol solutions, poor scalability, complicated purification methods as well as the generation of large amounts of waste, in part due to the need of neutralizing the produced lactate salts [20] , [21] . This issue of lactate formation and subsequent salt generation through neutralization is also common to all previous chemocatalyzed conversions of glycerol to LA and has been very recently circumvented by the synthesis of methyl lactate, instead of the lactate salts, in diluted methanol solutions of glycerol using a heterogeneous gold catalyst [22] . An important advantage of the fermentative route is the generation of enantiopure L -LA. Whereas the synthesis of green solvents and several commodity chemicals from LA does not have any chirality requirement, its polymerization to produce PLA requires enantiopure monomers to yield high-performance polyester with optimal thermal and mechanical properties. While 260,000 tons of LA are produced annually, the demand is projected to grow rapidly, necessitating a search for alternative methods of LA production [20] , [21] . Alternative chemoselective methods to produce LA, not only from glycerol, but also from other biomass-derived sources such as sugars and cellulose [20] , [23] , [24] , [25] , could offer advantages over current biological methods. An exploitable feature is that heterogeneous catalysts produce racemic LA that, after racemic resolution, could give access to D -LA, difficult to produce by fermentation. Previous chemocatalytic attempts have focused on the hydrogenolysis of aqueous glycerol solutions in alkaline media, but these reactions require high temperatures (180–200 °C) and high hydrogen pressures [26] , [27] , [28] , [29] . Chaudhari [30] and Pinel [31] , [32] independently demonstrated that a change in the atmosphere can increase the selectivity for LA, avoiding the need for hydrogen gas. In a remarkable and original approach, Liu and co-workers [33] employed Au-Pt/TiO 2 to catalyse the selective aerobic oxidation of glycerol to LA at low temperature (90 °C). However, all previous examples resulted in low LA productivities due to the low glycerol or sugar concentrations in the aqueous mixtures employed. In addition, the lack of homogeneous systems results in limited selectivity and makes it difficult to fully understand the reaction mechanisms and therefore pursue the rational design of new catalysts. Following our studies on iridium-mediated hydrogen-transfer reactions, we report the first homogeneous catalysts for the clean conversion of glycerol to LA with high efficiency and selectivity. Our system is also consistent with green chemistry principles (mild conditions, no solvent, reactions in air and so on). We have even been able to convert crude glycerol waste samples from a biodiesel refinery without previous purification. Catalyst screening and selectivity Glycerol is a highly functionalized molecule when compared with standard fossil hydrocarbon feedstocks. The three hydroxyl groups offer many possibilities for glycerol to act as a raw material for chemical synthesis. Conversion of glycerol to LA and H 2 is atom economic but requires both a redox and a dehydration/rehydration step. Typically, the metal-catalyzed dehydrogenation step yields either DHA or glyceraldehyde (GAL), which can then be converted into LA (in the form of lactate) under alkaline conditions ( Fig. 3 , vide infra ). To achieve high LA selectivities, side reactions such as C–C cleavage, overoxidation and overreduction must be minimized, a difficult task for those heterogeneous catalysts that operate under harsh conditions. Recently, Farnetti and co-workers [34] demonstrated the potential of homogeneous iridium catalysts for the acceptorless dehydrogenation of glycerol to DHA, albeit in low yields, while Peris and co-workers reported the potential of Ir-NHC catalysts (NHC= N -heterocylic carbene) for the reduction of carbonyl compounds using glycerol as solvent and hydrogen donor [35] , [36] . These results encouraged us to screen a small library of homogeneous Cp*Ir precatalysts (Cp*=η 5 -C 5 Me 5 ), including Ir-NHC species, that we previously employed in hydrogen-transfer catalysis [37] , [38] . We thought that carrying out dehydrogenation catalysis in the presence of a sufficient amount of base could be beneficial in: (i) promoting the dehydration/rehydration step towards the desired LA and (ii) trapping the LA as lactate salts, thus enhancing conversion and selectivity. 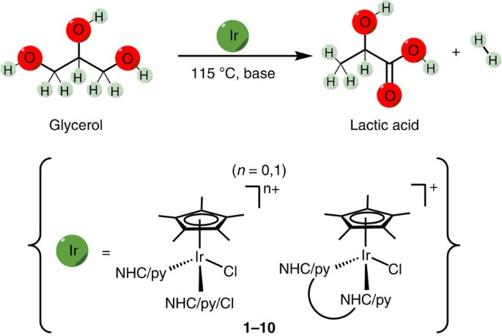Figure 1: Iridium-catalyzed conversion of glycerol to LA. The transformation and catalyst structures are shown. Figure 1: Iridium-catalyzed conversion of glycerol to LA. The transformation and catalyst structures are shown. 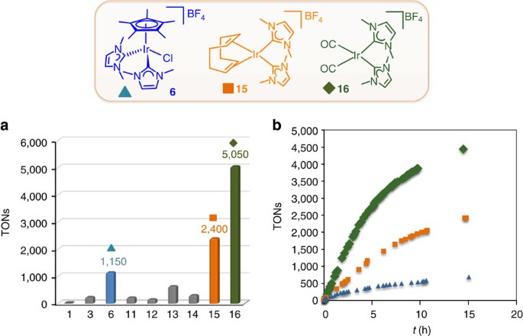Figure 2: Optimization of the iridium catalyst. (a) Activity of complexes1,3,6and11–16in the conversion of glycerol to LA, where1is [Cp*IrCl2]2,11is [Ir(COD)Cl]2,12is [Ir(CO)2Cl]2,13is [Ir(COD)(IMe)Cl] and14is [Ir(CO)2(IMe)Cl]. Conditions: 115 °C, 15 h, neat glycerol, 3 μmol Ir catalyst (0.007 mol%), KOH (8 M), N2. (b) Reaction profile by hydrogen evolution measurements with gas burette. Full size image Figure 2: Optimization of the iridium catalyst. ( a ) Activity of complexes 1 , 3 , 6 and 11–16 in the conversion of glycerol to LA, where 1 is [Cp*IrCl 2 ] 2 , 11 is [Ir(COD)Cl] 2 , 12 is [Ir(CO) 2 Cl] 2 , 13 is [Ir(COD)(IMe)Cl] and 14 is [Ir(CO) 2 (IMe)Cl]. Conditions: 115 °C, 15 h, neat glycerol, 3 μmol Ir catalyst (0.007 mol%), KOH (8 M), N 2 . ( b ) Reaction profile by hydrogen evolution measurements with gas burette. 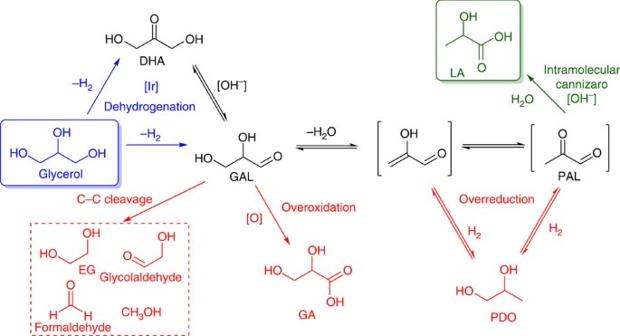Figure 3: Proposed mechanism for the conversion of glycerol to lactic (green) and other common byproducts (red). Products: DHA; GAL; EG; GA, glyceric acid; PDO; PAL; LA. Full size image Figure 3: Proposed mechanism for the conversion of glycerol to lactic (green) and other common byproducts (red). Products: DHA; GAL; EG; GA, glyceric acid; PDO; PAL; LA. Full size image A family of Cp*Ir complexes ( 1 – 10 in Supplementary Fig. 1 ) bearing a variety of ligands, both N- and C- based, neutral and anionic, chelating and monodentate ligands, was screened for the acceptorless dehydrogenation of neat glycerol to produce LA and H 2 ( Fig. 1 ; 0.007 mol% catalyst, 115 °C, 15 h, 8 M KOH (~0.6 equiv. with respect to glycerol)). In analogy to our previous studies, the bis-NHC precatalyst [Cp*Ir(IMe) 2 Cl] + BF 4 − ( 6 ) (IMe=1,3-dimethylimidazol-2-ylidene) exhibited the best catalytic performance, with a turnover number (TON; calculated as the molecules of LA produced per molecule of catalyst) of 1,150, whereas the other iridium species showed TONs between 20 and 60 ( Supplementary Fig. 2 ). Precatalyst [Cp*Ir(IMe)Cl 2 ] ( 3 ) also gave good results, with a TON of 242. No LA formation was detected in the absence of iridium precatalysts. It is noteworthy that hydrogen gas is liberated as a valuable side product in the course of the reaction (1 molecule of H 2 per molecule of LA) and can be collected from the headspace. Optimization of reaction conditions Encouraged by these results, we proceeded to optimize the reaction conditions with 6 ( Table 1 ). Potassium hydroxide appeared to be the best choice of base out of those tested (entries 1–4), probably due to its higher solubility in neat glycerol. Increasing the amount of base considerably speeds up product formation, whereas in its absence no conversion was recorded. To the best of our knowledge, this catalyst exhibits the highest selectivity for LA reported to date (≥95%). The best results were obtained with neat glycerol, likely due to intrinsic higher concentration, although the catalysis also works well in aqueous solutions (entries 11 and 12) without loss of selectivity. Interestingly, the reaction is somewhat tolerant of air (entries 13 and 14), an important aspect for practical application. Indeed, all our precatalysts can be stored under air without special precautions and show no sign of deactivation after several months. Increasing the temperature to 140 and 160 °C yielded the highest TONs, although at 160 °C we observed the appearance of small amounts of insoluble solids accompanied by a reduction in the mass balance to around 95%. Table 1 Optimization of reaction conditions. Full size table Iridium catalyst optimization In prior studies, we proposed that the remarkable activity of 6 in hydrogen-transfer catalysis could be attributed to catalyst preactivation by means of Cp* loss, opening up additional active sites on the catalyst. If so, the Cp* is unnecessary and precatalysts with other ancillary ligands might be good or even better. We prepared COD (1,5-cyclooctadiene) and bis-carbonyl Ir(I) complexes bearing two IMe ligands by common synthetic procedures (see Methods section for details). Indeed, switching from Cp* to COD in 15 doubled the catalytic activity (TON=2,400) under our standard reaction conditions, and, even better, the bis-carbonyl complex 16 yielded a TON of 5,050 ( Fig. 2a ). These values greatly surpass the activity of previously reported heterogeneous systems. The activity of precatalysts 6 , 15 and 16 was examined in greater detail by monitoring the evolution of H 2 using gas burette measurements ( Fig. 2b ; see Supplementary Fig. 12 ; Supplementary Methods ). For comparison, we prepared and assayed compounds 13 ([(COD)Ir(IMe)Cl]) and 14 ([(CO) 2 Ir(IMe)Cl]), each bearing a single NHC ligand. These species exhibited higher TONs than their Cp* analogue 3 , but complexes with two NHC ligands still showed the highest activities, so, as we proposed in prior work, we believe that both NHCs are retained by the metal during catalysis. Once more, the selectivity towards LA is ≥95% in all cases. Remarkably, while the activity of compound 15 partly degraded in the presence of air (1,750 TON, 73% of activity under nitrogen), compound 16 was equally active under nitrogen or in air (5,050 versus 5,045 TON, respectively). Homogeneity studies To check the homogeneous character of our catalysts, several experiments were carried out. First, it was determined that other, simpler forms of iridium, namely IrCl 3 , IrO 2 , Ir/C and freshly prepared Ir 0 nanoparticles (2–3 nm) exhibited much lower activities ( Supplementary Table 1 ) than the Ir(NHC) precatalysts. Next, poisoning experiments were undertaken with triphenylphosphine and mercury ( Supplementary Figs 2 and 3 ). On addition of triphenylphosphine, the activity of compounds 6 and 16 dramatically decreased, but the presence of mercury did not seem to affect their catalytic performance. While PPh 3 is expected to block needed sites at a homogeneous catalyst, Hg should block sites on a heterogeneous system [39] . Finally, after several experiments at 115 °C with higher catalyst loadings ( 15 , 16 ), no characteristic 1 H NMR resonances for free imidazolium salts were seen, whereas integration of the complicated set of aromatic signals due to ligated NHC groups matched the initial catalyst loading (internal standard). These results strongly suggest that in situ deligation of the molecular precursors to give heterogeneous materials does not account for the high activity observed [39] . Productivity optimization and application to crude glycerol After optimizing reaction conditions and iridium precursors and providing evidence against heterogeneous catalysis, our focus shifted to achieving higher LA productivities. Both biological fermentative processes and previously reported heterogeneous catalytic conversion of glycerol to LA give generally poor productivities harming their viability as industrially feasible methods. Ochoa-Gómez and co-workers [40] tackled the problem following a hydrothermal approach using up to 3.5 M glycerol concentrations, but this required temperatures as high as 280 °C. In our system, increasing the amount of KOH to 1.1 equiv. with respect to glycerol allowed us to achieve up to 94% conversion and 97% LA selectivity (see Table 2 , entry 2). The higher amount of base necessitated the addition of water for complete solubility. However, since one molecule of water is generated per lactate anion, conversions as high as 90% were achieved without additional solvent (entry 1). 1,2-propanediol (PDO), ethylene glycol (EG) and formic acid (FA) were identified as the major side products (2–4% overall) by 1 H NMR after addition of authentic standards. The amount of EG seems to remain constant over the reaction profile, whereas PDO and FA are more abundant at shorter times (entries 3–5). Reducing the catalyst loading to 20 p.p.m. allowed us to surpass 30,000 TON (entry 10), again with a LA selectivity of over 95%. Table 2 High productivities for LA using catalyst 16. Full size table In view of the remarkable productivity and LA selectivity achieved, we decided to test catalyst 16 with an authentic sample of glycerol derived from biodiesel production. The crude glycerol produced in typical biodiesel plants contains between 60 and 85 wt% glycerol [41] , as well as a plethora of impurities in quantities that make it difficult to use in most applications [42] . The high cost of crude glycerol purification [43] forces small and medium biodiesel producers to pay for its disposal and incineration, which has caused the price of crude glycerol to fall to zero or even below [42] . Direct conversion of crude glycerol by fermentative processes has been reported [44] , [45] , but only a limited number of microorganisms exhibit tolerance against the impurities present in the crude mixture [46] . Crude glycerol has been successfully employed for generating hydrogen and syngas, but chemical catalytic transformations into value-added products such as LA are lacking [47] . To our delight, catalyst 16 showed a decreased but still very satisfactory activity in converting crude glycerol (68% glycerol content) into LA under relatively mild conditions and with the same high selectivity as before. Conversion of 98% and LA selectivity of 96% were achieved using 0.6 mol% of 16 at 130 °C (mass balance 97%, see Supplementary Table 3 ). The process was scalable to 3 ml of crude glycerol with similar results. Mechanistic investigations We have been able to obtain some initial insights into the mechanism. In the absence of either iridium precursor or KOH, no LA (or other derivative) is detected under otherwise identical conditions as in Table 1 . Many of the common intermediates proposed in glycerol hydrogenolysis and oxidation are not stable at the high pH employed for catalysis, so several experiments were performed with lower base loadings. These experiments allowed for the identification of two species absent under more basic conditions, namely pyruvaldehyde (PAL) and acetol (from hydrogenation of PAL). Interestingly, these species were only identified when using catalysts 15 and 16 , and were not detected in reactions with 6 . When the common dehydrogenation products of glycerol, DHA and GAL were treated with aq. KOH (8 M, 115 °C), they readily converted into LA ( ca. 70 and 50%, respectively) and other unidentified species both in the presence and absence of iridium catalyst. Moreover, identical results were obtained for DHA and GAL under 1 atm of H 2 with and without iridium. Interestingly, when PDO was used as starting material under standard conditions with iridium, 3% conversion to LA was measured under H 2 (1 atm), while in the absence of iridium PDO remained unaltered. Finally, LA remained unchanged when subjected to standard conditions, with and without iridium catalyst. In light of these results, and previous investigations [26] , [27] , [28] , [29] , [30] , [31] , [32] , [33] , we tentatively propose that glycerol conversion may proceed through the mechanism depicted in Fig. 3 . The first step would be iridium-catalyzed dehydrogenation of glycerol to DHA or GAL, which are known to interconvert in alkaline media [48] , [49] . Previous homogeneous iridium catalysts have proven effective in the dehydrogenation of glycerol to DHA [34] , [35] , [36] and it is plausible to believe that our iridium precursors might be more selective for the dehydrogenation of the secondary alcohol to yield DHA over GAL, consistent with our observation that DHA led to higher yields of LA than GAL when used as starting material. Subsequent base-catalyzed dehydration of GAL would lead to PAL and its enol form, which reacts by an intramolecular Cannizaro reaction to yield LA [29] , [30] , [31] , [33] . The high selectivity exhibited by the present iridium precatalysts could be a result of blocking the three main side routes depicted in Fig. 3 , namely, overoxidation, overreduction and C–C cleavage. The major side product observed (<2%) is EG, which is probably produced from GAL by a retro-aldol reaction, with concomitant formation of FA [28] . Further iridium-catalyzed dehydrogenation of EG and FA would likely account for the different experimental ratios of these two side products under different reaction conditions. Overoxidation of GAL to glyceric acid has not been seen in this study. Interestingly, the reduction of PAL to PDO (also evidenced by the observation of acetol at lower base loadings) is partly reversible due to iridium-catalyzed dehydrogenation, which, along with the irreversibility of LA formation, might help account for the remarkable selectivity achieved. Finally, preliminary investigations were carried out to assess the nature of the active catalytic species. Complex mixtures of iridium hydride signals were recorded by 1 H NMR spectroscopy between −5 and −24 p.p.m. after standard catalytic runs using 6 , 15 and 16 ( Supplementary Fig. 4 ). Reaction of 16 with KOH (10–15 equiv.) in methanol solutions also resulted in complex hydridic regions by 1 H NMR, with several resonances in common with catalysis experiments. Two-dimensional NMR analysis revealed the formation of mono- and polyhydride species for compounds 15 and 16 ( Supplementary Figs 5–7 ). High-resolution mass spectroscopy (HRMS) analysis (Fourier transform ion cyclotron resonance (FT-ICR)) allowed for the identification of monomeric and dimeric iridium complexes containing two or three NHC ligands per iridium, up to two metal hydrides and one or no carbon monoxide fragments ( Supplementary Figs 8–11 ). After numerous attempts, two iridium species ( 17 and 18 ) formed under standard reaction conditions were isolated in low yields (~5–10%) and characterized by spectroscopic techniques and X-ray diffraction studies ( Fig. 4 ; Supplementary Fig. 13 ; Supplementary Tables 5–7 ). Compounds 17 and 18 contain three NHC ligands per iridium atom, as well as two metal hydrides. Compound 17 is dinuclear and displays two terminal and two bridging metal hydrides, whereas compound 18 is mononuclear and has one carbonyl ligand. This constitutes a rare example of such a ligand rearrangement [50] , [51] , since NHCs are typically believed to be tightly bound to the metal centre [52] . Complex 17 showed a low TON of 40 under standard catalytic conditions (0.007 mol%, KOH 8 M, 15 h, 115 °C), identifying it as a product of catalyst deactivation rather than an active species. Unfortunately, compound 18 decomposed under inert atmosphere before we were able to assess its catalytic potential and all attempts to isolate it again proved unsuccessful. 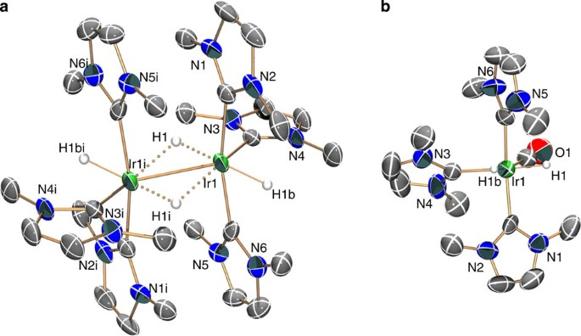Figure 4: Oak Ridge Thermal Ellipsoid Plot diagrams of the cationic portions of compounds17(panel a) and18(panel b). 50% thermal ellipsoids are shown. Hydrogen atoms (except iridium hydrides) and solvent molecules have been omitted for clarity. To further investigate the role of NHC reorganization, several catalytic experiments were performed with additional equivalents of [1,3-dimethylimidazolium]BF 4 ( Supplementary Table 4 ). Whereas addition of one extra equivalent of the NHC precursor increased the catalytic activity of mono-NHC complexes 13 and 14 , it had little effect when added to bis-NHC species 15 and 16 . These findings suggest that the chemistry taking place under catalytic conditions with regards to the active catalyst is certainly much more complicated than commonly expected and likely includes the formation of complex mixtures of iridium hydride and polyhydride species, as well as unusual NHC reorganization processes. Experimental results clearly indicate that two NHCs are pivotal for high catalytic turnover, an idea that will be pursued in future investigations. Figure 4: Oak Ridge Thermal Ellipsoid Plot diagrams of the cationic portions of compounds 17 (panel a) and 18 (panel b). 50% thermal ellipsoids are shown. Hydrogen atoms (except iridium hydrides) and solvent molecules have been omitted for clarity. Full size image The catalytic transformation of biomass-based feedstocks into useful chemicals of all kinds has grown enormously in the last two decades [3] , [53] . Although there are several examples of well-defined homogeneous catalysts for these conversions, the majority of systems are based on heterogeneous platforms, which generally offer higher robustness and applicability under the harsh conditions required to upgrade raw materials such as lignin, cellulose or even glycerol. The conversion of glycerol to LA is a classic example, and the catalysts reported here constitute the first homogeneous systems reported for this transformation. When compared with heterogeneous catalysts, the activity and especially the selectivity exhibited by homogeneous catalysts are frequently easier to tune by rational modification of the ligand environment. Under the experimental conditions employed in this work, our iridium precursors gave selectivities higher than 95% for LA, the highest reported to date for any chemocatalyzed processes and more typical of fermentative processes. Besides their high selectivity, an additional advantage of fermentative routes from sugars is the production of enantiopure L -LA. This is of paramount importance for the synthesis of PLA (although not required for most of the other LA applications), since enantiopure L -LA (or D -LA) yields the desired high-quality PLA, having improved thermal and mechanical properties with respect to amorphous PLA obtained from racemic LA [54] . However, recent studies revealed that the combination of enantiopure L -PLA and D -PLA (1:1 ratio) leads to stereocomplexed PLA, with greatly enhanced properties compared with their stereopure polymer forms [55] , [56] . The availability of D -PLA is still very limited and its price too high for many applications. Although several organisms are capable of producing D -LA [57] , [58] , [59] , its production level is still very low and its potential for scalability seems poor. Chemocatalyzed processes such as the one reported here allow access to D -LA in the racemic mixtures, which could plausibly be isolated by racemic resolution or by enzymatic degradation of the L -LA form, and thus offer potential pathways to cheaper D -LA [60] , [61] , [62] , [63] . Another contribution of this work is the production of hydrogen gas as a valuable side product. Previous heterogeneous systems for this transformation typically required hydrogen [26] , [27] , [28] or oxygen [33] inputs to follow the hydrogenolysis or oxidative dehydrogenation pathways, respectively. Our initial iridium-mediated acceptorless dehydrogenation step allows for the generation of hydrogen gas that could be employed elsewhere in a commercial plant, reducing the overall cost of the process. Finally, our mechanistic investigations have identified several catalyst deactivation products. This opens the way to further optimization of these and related catalysts by ligand modification to increase their stability and activity. In summary, we have synthesized the first homogeneous catalysts for the conversion of glycerol to LA. The iridium catalysts tested here exhibit the highest activity for this transformation reported to date, with TONs at least one order of magnitude over that of the current best heterogeneous systems. Our method fulfills the main principles of green chemistry: mild conditions, no solvent required, renewable feedstock, degradable product and catalyst loadings as low as 0.003 mol%. It can be applied to crude glycerol samples derived from the biodiesel industry without previous pretreatment or purification. This could much reduce the costs of upgrading glycerol and makes the process environmentally sound. The use of neat glycerol enhances LA productivity beyond previous limits for fermentation or heterogeneous catalytic routes. These results provide guidance for further development of more effective catalysts, ideally based on non-precious metals, for this and other biomass-related transformations. General experimental details NMR spectra were recorded on Agilent DD2-400, -500 or Bruker AMX-500 spectrometers at ambient probe temperatures ( Supplementary Figs 14–18 ). Chemical shifts are reported with respect to residual internal protio solvent for 1 H and 13 C{ 1 H} NMR spectra. The chemical shift δ is reported in units of p.p.m. Mass spectrometry analyses were performed by the Mass Spectrometry and Proteomics Resource of the W.M. Keck Foundation Biotechnology Resource Laboratory at Yale University. Fourier transform infrared (FTIR) spectra were recorded in a Thermo Nicolet 6700 equipped with a diamond attenuated total reflectance cell. General procedure for conversion of glycerol to LA To a reactor vessel (Radleys Carousel 12 Place Reaction Station, RR98030) or Schlenk tube coupled to a condenser and equipped with a stir bar was added the corresponding iridium catalyst (0.003–0.03 mol%) and potassium hydroxide (0.58–1.1 equiv. versus glycerol). The flask was charged with previously deoxygenated glycerol (1.5–3 ml) under nitrogen atmosphere. For reactions with 1.1 equiv. of KOH, deoxygenated water (0.1–0.5 ml) was also added. The reaction was heated to 70–160 °C for 15–24 h, then the vessel removed from heat and deuterium oxide (2 ml) and an aqueous solution of sodium acetate (internal standard) immediately added to the thick reaction mixture with stirring. Conversion and selectivity were obtained by 1 H NMR analysis of the crude mixtures ( Supplementary Fig. 19 ). Compound 15 This complex was synthesized based on a previously reported procedure [64] . [Ir(COD)Cl] 2 (200 mg, 0.298 mmol) and Ag(IMe) 2 BF 4 (250 mg, 0.648 mmol) were added to a 100-ml round bottom Schlenk flask with a magnetic stir bar. The Schlenk was evacuated and purged with dry nitrogen. Dry dichloromethane (20 ml) was added under nitrogen and the mixture stirred at room temperature for 3 h in the absence of light. The resulting dark orange solution was run through a short silica plug in air. A bright orange band was collected by flushing the silica with acetone, leaving behind a darker orange/brown band. The solvent of the combined product fractions was removed under reduced pressure and the solid taken back in minimal dichloromethane. The product was precipitated by the addition of diethyl ether and collected by filtration to yield a bright orange powder (252 mg, 73% yield). 1 H NMR (600 MHz, CD 2 Cl 2 ): δ 6.97 (s, 2H), 3.89 (s, 6H), 3.82 (s, 2H), 2.34–2.20 (m, 2H), 2.00–1.90 (m, 2H). 13 C{ 1 H} NMR (151 MHz, CD 2 Cl 2 ): δ =177.93 (s), 123.25 (s), 76.75 (s), 38.34 (s), 31.81 (s). HRMS (FT-ICR, m / z ): [M] + calcd. for C 18 H 28 IrN 4 , 493.1943; found, 493.1901. Compound 16 [Ir(COD)(IMe) 2 ]BF 4 ( 15 , 50 mg, 0.0862, mmol) was added to a 100-ml round bottom Schlenk flask with a magnetic stir bar. The Schlenk was evacuated and purged with carbon monoxide. Dry dichloromethane (2 ml) was added under CO atmosphere and the vessel sealed and stirred at room temperature for 1 h. The solution visibly turned from orange to yellow within minutes. The solvent was reduced to 5 ml under reduced pressure and diethyl ether was added to precipitate a vibrant yellow powder, which was collected by filtration (40 mg, 87% yield). 1 H NMR (600 MHz, CD 2 Cl 2 ): δ =7.12 (s, 1H), 3.69 (s, 3H). 13 C{ 1 H} NMR (151 MHz, CD 2 Cl 2 ): δ 180.60 (s), 124.42 (s), 110.54 (s), 38.58 (s). HRMS (FT-ICR, m / z ): [M] + calcd. for C 12 H 16 IrN 4 O 2 , 441.0902; found, 441.0870. FTIR (solid): ν (CO)=1,995, 2,060 cm −1 . How to cite this article: Sharninghausen, L. S. et al . Efficient selective and atom economic catalytic conversion of glycerol to lactic acid. Nat. Commun. 5:5084 doi: 10.1038/ncomms6084 (2014). Accession codes: The X-ray crystallographic coordinates for structures reported in this Article have been deposited at the Cambridge Crystallographic Data Centre (CCDC), under deposition numbers CCDC 993919 ( 16 ), 993920 ( 17 ) and 993921 ( 18 )). These data can be obtained free of charge from The Cambridge Crystallographic Data Centre via www.ccdc.cam.ac.uk/data_request/cif .